Mitotic cell rounding and epithelial thinning regulate lumen growth and shape Many organ functions rely on epithelial cavities with particular shapes. Morphogenetic anomalies in these cavities lead to kidney, brain or inner ear diseases. Despite their relevance, the mechanisms regulating lumen dimensions are poorly understood. Here, we perform live imaging of zebrafish inner ear development and quantitatively analyse the dynamics of lumen growth in 3D. Using genetic, chemical and mechanical interferences, we identify two new morphogenetic mechanisms underlying anisotropic lumen growth. The first mechanism involves thinning of the epithelium as the cells change their shape and lose fluids in concert with expansion of the cavity, suggesting an intra-organ fluid redistribution process. In the second mechanism, revealed by laser microsurgery experiments, mitotic rounding cells apicobasally contract the epithelium and mechanically contribute to expansion of the lumen. Since these mechanisms are axis specific, they not only regulate lumen growth but also the shape of the cavity. Defects in lumenogenesis cause severe diseases such as polycystic kidney disease, brain ventricle closure anomalies or deafness associated with vestibular aqueduct enlargement [1] , [2] , [3] . The morphogenetic mechanisms of lumen growth have recently been analysed, with most of the studies focusing on tubular organs [4] , [5] , [6] . However, many organs have cavities with elaborate shapes adapted to their function, such as the heart, the brain and the inner ear. How the epithelium directs the growth of a lumen with geometrical asymmetries to generate a particular three-dimensional (3D) shape is still unknown. Lumen formation is initiated either by invagination of the epithelium, by hollowing mechanisms in which opposed apical surfaces are separated by the secretion of extracellular matrix and fluid, or by cavitation in which loss of cells inside the organ generates a new space [7] . The acquisition of apicobasal (ab) polarity seems to be a shared feature in all cavity-forming processes, while other aspects such cell proliferation, secretion of repulsive molecules or cell rearrangements are particular to each cavity [8] . Lumen growth requires coordination between fluid ingress and increase of the luminal epithelial surface area. Fluids ingress has been shown to rely on a functional Na + /K + ATPase pump, the CFTR chloride channel and the formation of both paracellular pores and barriers by claudin proteins [5] , [9] , [10] , [11] . The present view of the process indicates that fluid ingress is mediated by transepithelial fluid transport, in which the epithelium is considered as a pump driving fluid movement from outside of the organ into the lumen [12] , [13] , [14] . Remarkably, although this epithelium is also a fluid-filled structure, the exact contribution of intraepithelial fluid to lumen morphogenesis is unclear. The epithelial wall adapts to enable the growth of the lumen via various rearrangements of the tissue [8] . Cell division plays an essential role by increasing the number of cells forming the epithelial layer, as described in mammalian vasculature and kidney [4] , [14] . During neural tube morphogenesis, oriented cell division also contributes to lumenogenesis [15] . The epithelial surface area can also increase independently of cell division, but by remodelling cell shape, as shown during Drosophila tracheal morphogenesis. In this case, anisotropic increase of the apical cell surface drives tracheal dorsal trunk elongation [16] , while in tracheal branches the tube is elongated by cell intercalation [6] . Here we use zebrafish inner ear morphogenesis to analyse the growth mechanisms determining lumen dimensions, as the small and superficial lumen of the otic vesicle is radially asymmetric and growth can be visualized in vivo . Inner ear morphogenesis begins when the otic placode develops from a thickening of the ectoderm adjacent to the hindbrain [17] . Then the otic primordium grows into a solid mass of cells in which a central lumen appears and expands to form the otic vesicle [17] . Subsequently, the lumen subdivides and the inner ear acquires its highly elaborate adult shape [18] . While some mechanisms that build the complex late inner ear shape were identified [19] , the early morphogenetic events leading to lumen formation and expansion were not explored. We quantitatively analyse the lumenogenesis dynamics of the zebrafish inner ear by high-resolution four-dimensional (4D) live imaging. We uncover new morphogenetic mechanisms driving the growth and shape of the lumen. First, we find asymmetric fluid loss of the epithelial cells that parallels the expansion of dorsoventral (DV) and mediolateral (ML) axes, thinning the epithelium. This remodelling process seems to create new luminal space and cause a net redistribution of fluids within the organ from the epithelial cells to the lumen, highlighting a role of intraepithelial fluids in lumen expansion. Second, we show that the length of the anteroposterior (AP) axis is finely tuned by a mechanical mechanism driven by mitotic cells. We identify mitotic rounded cells exerting a pulling force over the luminal surface of the epithelium, a direct mechanic effect of individual cells to expand the lumen. These axis-specific mechanisms shape the lumen during expansion. Zebrafish inner ear lumen forms by cord hollowing To analyse the dynamics of inner ear lumen formation in zebrafish, we used high-resolution 4D confocal imaging. The ear primordium is evident from 13 h.p.f. (hours post fertilization) as a distinguishable oval structure ( Fig. 1a ; Supplementary Movie 1 ). While epithelialization is already visible in the medial side of the vesicle adjacent to the hindbrain, the lateral side remains unorganized, acquiring its defined epithelial structure upon lumen formation. Luminal space is clearly visible at 16.5 h.p.f., when two small unconnected lumens arise. At 17 h.p.f., these two lumens fuse into a single bigger slit-shaped lumen, and thereafter the cavity expands ( Fig. 1a ). 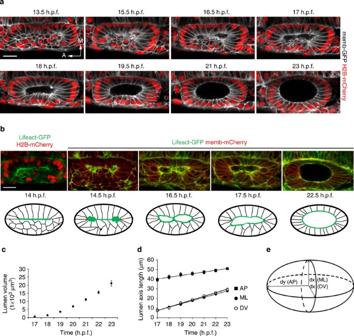Figure 1: Inner ear hollowing dynamics. (a) Dorsal confocal live imaging of otic vesicle from 13.5 to 23 h.p.f. showing lumen formation and expansion in coronal planes. Membranes and nuclei are stained by co-injection of membrane-GFP and H2B-mCherry mRNAs, respectively. Scale bar, 20 μm. (b) Dynamics of F-actin-polarized distribution during lumen formation and expansion. Embryos are Tg(actb1:lifeact-GFP). Schematic representations of F-actin localization are shown below (F-actin in green, membranes in black). Scale bar, 20 μm. (c,d) Quantification of lumen volume (c) and length of each axis (d) during expansion of the cavity, obtained from data acquisition of 4D movies. Data are mean±s.e.m. (n=5). In (d), a linear regression for the data for each axis is shown.r=0.98 (AP) and 0.99 (ML and DV). (e) 3D lumen drawing showing its biaxial ellipsoidal shape at 23 h.p.f. The radii of the AP, ML and DV axes are shown. Figure 1: Inner ear hollowing dynamics. ( a ) Dorsal confocal live imaging of otic vesicle from 13.5 to 23 h.p.f. showing lumen formation and expansion in coronal planes. Membranes and nuclei are stained by co-injection of membrane-GFP and H2B-mCherry mRNAs, respectively. Scale bar, 20 μm. ( b ) Dynamics of F-actin-polarized distribution during lumen formation and expansion. Embryos are Tg(actb1:lifeact-GFP). Schematic representations of F-actin localization are shown below (F-actin in green, membranes in black). Scale bar, 20 μm. ( c , d ) Quantification of lumen volume ( c ) and length of each axis ( d ) during expansion of the cavity, obtained from data acquisition of 4D movies. Data are mean±s.e.m. ( n =5). In ( d ), a linear regression for the data for each axis is shown. r =0.98 (AP) and 0.99 (ML and DV). ( e ) 3D lumen drawing showing its biaxial ellipsoidal shape at 23 h.p.f. The radii of the AP, ML and DV axes are shown. Full size image Time-lapse imaging of Lifeact tagged to green fluorescent protein (GFP) [20] allowed us to observe that at 14 h.p.f., the epithelium is already polarized and displays a stripe of apical F-actin accumulation in the tissue midline ( Fig. 1b ), delineating the surface where the lumen will develop. At 14.5 h.p.f., two poles enriched with F-actin appear at the extremes of the medial apical stripe. As the lumens form and coalesce into one, F-actin remains localized at the apical membrane ( Fig. 1b and Supplementary Fig. 1f ; Supplementary Movie 2 , see also Supplementary Fig. 1a–e for the localization of the polarity marker Pard3 and the cell junction protein ZO-1). On the basis of the above data, we define a lumen-assembly phase (from 13 to 17 h.p.f.) and a lumen expansion phase (from 17 to 23 h.p.f.). The growth of the lumen is anisotropic To better characterize how the geometric shape of the lumen is established during the expansion phase, we performed a quantitative analysis of dynamic changes in the dimensions at the organ, tissue and cellular level. We first analysed the kinetics of increase in lumen volume and observed that the expansion rate increases with time (mean volume expansion rate=3.4±0.3 × 10 3 μm 3 h −1 , Fig. 1c ). We then measured the length of the lumen axes during expansion. At 17 h.p.f., the lumen is slit shaped, with a long AP axis and short ML and DV axes of equal length ( Fig. 1a,d ). Interestingly, during the expansion phase, the growth of the axes of the lumen is anisotropic—the two short axes expand with similar and faster kinetics than the AP axis (axis expansion rate: ML=3.36±0.29 μm h −1 ; DV=3.72±0.39 μm h −1 ; AP=1.80±0.16 μm h −1 ; ML or DV versus AP P <0.01, t -test; Fig. 1d ). Thus, the main contribution to volume increase comes from growth of the lumen on the ML and DV short axes. At 23 h.p.f., the shape of the lumen approaches that of a biaxial ellipsoid ( Fig. 1e , Supplementary Fig. 1g,h ): an ellipsoid with one major axis (AP), and two minor axes of equal length (ML and DV; considering the similar dimensions and behaviour of these two axes, hereafter we will refer to the ML, meaning the analysis of both). In subsequent experiments, we aimed to unravel the morphogenetic mechanisms that establish the dimensions of the ellipsoid. Gross AP axis lumen length is determined before hollowing We have shown that the main expansion occurs along the ML axis and that the difference in the length between axes is already present before the expansion phase begins, which suggests that the gross length of the future AP axis might be established before the lumen opens. This could be a consequence of how the tissue is assembled during epithelialization. We reasoned that the AP length of the apical stripe at the midline, the structure that gives rise to the lumen, could be the main determinant of the future length of the AP lumen axis ( Fig. 2a ). To test this hypothesis, we reduced the length of the apical midline by decreasing the number of cells contributing to the organ primordium. We inhibited proliferation before the lumen starts to form, including the moment when the apical midline is assembling, but allowed proliferation to proceed normally thereafter so as not to interfere with the expansion phase. We used two distinct approaches to block cell proliferation—injection of an emi1 (early mitotic inhibitor 1) morpholino ( emi1 MO, effective only between 6 and 12 h.p.f. as previously reported [21] ); and incubation with a combination of aphidicolin and hydroxyurea (AH) [21] , [22] from 10 to 14 h.p.f. (95±1% of cell division events inhibited). At 14 h.p.f., the length of the apical stripe was reduced in comparison with that of the control embryos (length ratio emi1 MO/controlMO=0.74±0.04; AH/DMSO (dimethylsulphoxide)=0.77±0.02; Fig. 2b,c ). Interestingly, expansion in these embryos led to lumens with reduced AP length (length ratio emi1 MO/controlMO=0.64±0.04; AH/DMSO=0.57±0.02; Fig. 2b,c and Supplementary Movie 3 ) and normal ML length (length ratio emi1 MO/controlMO=1.01±0.05; AH/DMSO=1.05±0.04). Consistent with our hypothesis, the lumen displayed an abnormal shape, approaching a sphere instead of a biaxial ellipsoid ( Fig. 2b ) and the radial asymmetry was reduced (as indicated by the ratio between the AP and ML length (DMSO=2.29±0.09; controlMO=2.36±0.12; emi1 MO=1.53±0.06; AH=1.26±0.06; Fig. 2d )). Thus, we found that AP axis lumen length is primarily determined before the lumen opens and depends on the size of the apical domain of the tissue assembled during epithelialization. 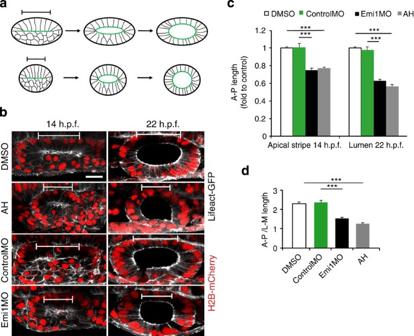Figure 2: Apical midline length determines gross AP lumen length. (a) Schematic representation of the influence of apical midline (green) length on later AP lumen length and shape. Segments highlight the different lengths of the initial apical stripe. (b) Confocal images of DMSO- or AH-treated andemi1MO or controlMO morphant embryos at 14 and 22 h.p.f. All embryos are Tg(actb1:lifeact-GFP). Segments show the AP length of the apical midline (14 h.p.f.) or the lumen (22 h.p.f.). Scale bar, 20 μm. (c) Fold change in AP length of the apical stripe at 14 h.p.f. and the lumen at 22 h.p.f. in DMSO- or AH-treated andemi1MO or controlMO morphant embryos. All values were related to DMSO. Data are mean±s.e.m. (n=8), ANOVA, ***P<0.001. (d) Quantification of changes in the ratio of AP to ML lumen length at 22 h.p.f. As ratio values approach 1, the shape of the lumen area in the images approaches that of a circle. Data are mean±s.e.m. (n=5), ANOVA, ***P<0.001. Figure 2: Apical midline length determines gross AP lumen length. ( a ) Schematic representation of the influence of apical midline (green) length on later AP lumen length and shape. Segments highlight the different lengths of the initial apical stripe. ( b ) Confocal images of DMSO- or AH-treated and emi1 MO or controlMO morphant embryos at 14 and 22 h.p.f. All embryos are Tg(actb1:lifeact-GFP). Segments show the AP length of the apical midline (14 h.p.f.) or the lumen (22 h.p.f.). Scale bar, 20 μm. ( c ) Fold change in AP length of the apical stripe at 14 h.p.f. and the lumen at 22 h.p.f. in DMSO- or AH-treated and emi1 MO or controlMO morphant embryos. All values were related to DMSO. Data are mean±s.e.m. ( n =8), ANOVA, *** P <0.001. ( d ) Quantification of changes in the ratio of AP to ML lumen length at 22 h.p.f. As ratio values approach 1, the shape of the lumen area in the images approaches that of a circle. Data are mean±s.e.m. ( n =5), ANOVA, *** P <0.001. Full size image Role of intraepithelial fluids in lumen expansion Since growth of the lumen is anisotropic, it also influences the shape of the lumen during expansion. We explored the cellular mechanisms responsible for this anisotropic growth. While the relevance of fluid movement in increasing the size of the cavity has been demonstrated in several experimental models [5] , [10] , [11] , with the involvement of paracellular transportation and epithelial chloride secretion [9] , [23] , its role in shaping the lumen has still not been evaluated. It is widely assumed that the increased intraluminal concentration of chloride (and other ions) promotes the movement of water from outside the organ into the lumen (by paracellular or transcellular transport), similar to what occurs in secretory epithelial organs [12] , [13] . Thus, this transepithelial transportation is thought to be what drives lumen growth. However, do the epithelia of lumen forming organs transport fluids only from one side of the tissue layer to the other? We noticed that the epithelium thins as the lumen grows ( Fig. 3a,b,g ). Since the otic epithelium is a monolayer of cells, thinning involves a reduction in the ab length of their lateral membranes ( Fig. 3f ). Therefore, it is possible that some of the luminal fluid could be fluid lost by epithelial cells. We measured in vivo the volume of individual cells in the otic vesicle at different time points during expansion. To this aim, we generated mosaic embryos expressing cytosolic GFP (or photoconverted kaede protein) and tracked different cells over time, imaging them at high spatial resolution for 3D reconstruction ( Fig. 3h and Supplementary Fig. 2a ). In 23-h.p.f. lumen-expanded vesicles, the volume of each tracked cell is smaller than its own at 17 h.p.f. (volume loss from 17 to 23 h.p.f., medial cell=29.67±2.94%, lateral cell=31.21±5.74%, anterior cell=18.61±2.14%, posterior cell=17.53±3.15%; Fig. 3i ), demonstrating that cells lose fluid during lumen growth. Thus, the widespread term of ‘organ inflation’ ( Fig. 3j ) in which the total size of the organ increases as fluids ingress into the lumen would not represent a complete view of the process. Alternatively, cellular fluid loss during epithelial thinning could also contribute to lumen expansion ( Fig. 3j ), without a substantial increase in the total size of the organ. In fact, there is only a small increase in the overall otic vesicle size during expansion, measured by their axes length ( Fig. 3k ). Furthermore, from 17 to 23 h.p.f., lumen volume increases more than double the otic vesicle volume (net increase in volume, lumen=20.4±1.6 × 10 3 μm 3 , vesicle=10.0±0.8 × 10 3 μm 3 ; P <0.005 t -test; Fig. 3l ). This implies that the epithelial tissue volume decreases during expansion, suggesting that ∼ 50% of the lumen volume at 23 h.p.f. was previously epithelial volume, and that the lumen grows at the expense of the epithelial volume. Interestingly, thinning of the epithelium during lumen growth does not seem to be specific to the inner ear, as we also observe it in the hindbrain during brain ventricle lumen growth ( Supplementary Fig. 2d–f ). 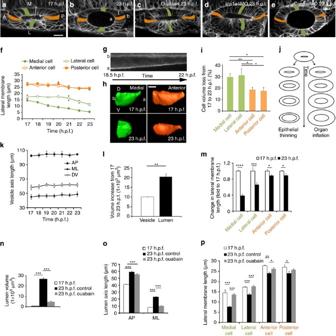Figure 3: Role of intraepithelial fluids in lumen expansion. (a,b) 17 and 23 h.p.f. otic vesicles of wt embryos expressing memb-GFP. Medial (M) and lateral (L) cells are depicted in green, anterior (A) and posterior (P) in orange. In (b), location of the various membrane domains are shown a, apical, b, basal and l, lateral. Scale bar, 20 μm. (c) Otic vesicle at 23 h.p.f. from an ouabain-treated embryo from 17 to 23 h.p.f. (d,e) Otic vesicle at 23 h.p.f. from anatp1a1MO- (d) or controlMO-injected (e) embryos. (f) Lateral membrane length over time plotted for cells located in different positions (n=12 cells, 5 embryos). (g) Kymograph of the medial epithelium from a time-lapse movie of lumen expansion in a wt embryo (white bar inadepicts the region used to generate the kymograph). a, apical; b, basal. (h) 3D reconstruction of an anterior (orange) and a medial (green) cell at 17 and 23 h.p.f. tracked in GFP mosaic embryos. Scale bar, 5 μm. (i) Cell volume loss from 3D reconstructed tracked cells located in various domains of the vesicle (n=15 cells in every position, 25 embryos). (j) Two models of lumen growth. On the left, the vesicle does not grow during lumen expansion, the fluid redistributes from the cells to the lumen, leading to a thinning of the epithelium. On the right, the fluids ingress to the lumen from outside of the organ and the thickness of the epithelium is maintained during expansion, increasing the size of the vesicle. (k) Length of the otic vesicle axes during expansion (n=5 embryos). (l) Volume increase of the lumen and vesicle during expansion (n=3 embryos). (m) Fold change of lateral membrane length (n=12 cells, 5 embryos). (n,o) Lumen volume (n) and lumen axis length (o) in control and ouabain-treated embryos at the times indicated (n=5). (p) Lateral membrane length at the times indicated in control and ouabain-treated embryos (n=12 cells, five embryos). Data are mean±s.e.m. ANOVA (n–p) ort-test (i,l,m). ****P<0.0001, ***P<0.001, **P<0.01 and *P<0.05. Figure 3: Role of intraepithelial fluids in lumen expansion. ( a , b ) 17 and 23 h.p.f. otic vesicles of wt embryos expressing memb-GFP. Medial (M) and lateral (L) cells are depicted in green, anterior (A) and posterior (P) in orange. In ( b ), location of the various membrane domains are shown a, apical, b, basal and l, lateral. Scale bar, 20 μm. ( c ) Otic vesicle at 23 h.p.f. from an ouabain-treated embryo from 17 to 23 h.p.f. ( d,e ) Otic vesicle at 23 h.p.f. from an atp1a1 MO- ( d ) or controlMO-injected ( e ) embryos. ( f ) Lateral membrane length over time plotted for cells located in different positions ( n =12 cells, 5 embryos). ( g ) Kymograph of the medial epithelium from a time-lapse movie of lumen expansion in a wt embryo (white bar in a depicts the region used to generate the kymograph). a, apical; b, basal. ( h ) 3D reconstruction of an anterior (orange) and a medial (green) cell at 17 and 23 h.p.f. tracked in GFP mosaic embryos. Scale bar, 5 μm. ( i ) Cell volume loss from 3D reconstructed tracked cells located in various domains of the vesicle ( n =15 cells in every position, 25 embryos). ( j ) Two models of lumen growth. On the left, the vesicle does not grow during lumen expansion, the fluid redistributes from the cells to the lumen, leading to a thinning of the epithelium. On the right, the fluids ingress to the lumen from outside of the organ and the thickness of the epithelium is maintained during expansion, increasing the size of the vesicle. ( k ) Length of the otic vesicle axes during expansion ( n =5 embryos). ( l ) Volume increase of the lumen and vesicle during expansion ( n =3 embryos). ( m ) Fold change of lateral membrane length ( n =12 cells, 5 embryos). ( n , o ) Lumen volume ( n ) and lumen axis length ( o ) in control and ouabain-treated embryos at the times indicated ( n =5). ( p ) Lateral membrane length at the times indicated in control and ouabain-treated embryos ( n =12 cells, five embryos). Data are mean±s.e.m. ANOVA ( n – p ) or t -test ( i , l , m ). **** P <0.0001, *** P <0.001, ** P <0.01 and * P <0.05. Full size image We also observed that the epithelial thinning is non-uniform, since both ab shortening and the fluid loss from cells located on the medial and lateral sides of the vesicle are more pronounced than that in anterior and posterior cells ( Fig. 3a,b,i,m ). Concomitant with the ab shortening, medial and lateral cells remodel and change their shape ( Fig. 3a,b,h and Supplementary Fig. 2b ). In contrast, the anterior and posterior cells maintain an ab elongated shape during lumen expansion ( Fig. 3a,b,h and Supplementary Fig. 2b ). Thus, changes in the morphology and volume of the cells are correlated in time and space with lengthening of the lumen axes (the lumen grows more in the ML axis), suggesting that the thinning process is related to the anisotropic growth of the axes. Next we directly evaluated the contribution of fluid movement to lumen expansion by incubating the embryos from 17 to 23 h.p.f. with ouabain, an inhibitor of the Na + /K + ATPase pump. This treatment disrupts transmembrane Na + and K + gradients, blocking ion flow and the consequent water displacement, resulting in inhibited fluid movement [9] , [10] . In agreement with what has previously been described for other lumens [9] , [10] , ouabain inhibits inner ear lumen growth ( Fig. 3c,n ). Interestingly, while ML expansion was blocked completely, AP expansion was only slightly reduced, resulting in an elongated slit shaped cavity ( Fig. 3c,o ). These results demonstrate that fluid movement is essential for normal ML expansion, and suggest that other mechanisms also operate to extend the AP axis. Concomitant with a defect in lumen growth, ouabain treatment also blocked the epithelial thinning events described above ( Fig. 3c,p and Supplementary Fig. 2c ), which functionally links ab cell shortening to fluid movement. Apical localization of both Pard3 and hZO1 was indistinguishable in treated and untreated embryos, suggesting that the ouabain phenotype is not caused by cell polarity or adhesion defects ( Supplementary Fig. 3 ). The phenotype of ouabain-treated embryos was reproduced by blocking the expression of the alpha subunit of the Na/K-ATPase pump by morpholino injection ( atp1a1 MO) [24] ( Fig. 3d ). Taken together, quantitative and functional data on cellular volume and cell remodelling dynamics are consistent with the presence of an epithelial thinning mechanism that would redistribute fluids within the organ to promote lumen growth. Since this thinning process is not uniform, it could also contribute to shape the cavity. Local epithelial contraction during mitotic cell rounding Since fluid movement does not seem to be the main driver of the AP growth, we explored other cellular mechanisms contributing to AP expansion. Cell division is important for lumen growth in different organs [7] . This led us to explore in detail the process of cell division during expansion by high temporal resolution 4D live imaging. We observed that the nuclei migrate to the apical epithelial surface to divide (an interkinetic nuclear migration hallmark of many neuroepithelial tissues; Fig. 4a,b and Supplementary Movie 4 ) and then the cell begins to change its shape as part of mitotic cell rounding ( Fig. 4a,b ). Later, cytokinesis proceeds and every nucleus returns to the basal domain. Notably, some of these mitotic events were associated with a local contraction of the epithelium ( Fig. 4b ; Supplementary Movie 5 ), in particular those located within or relatively close to the anterior and posterior vertices of the vesicle. This contraction can be observed as a decrease in the ab length of the epithelium ( Fig. 4b–d,f ; Supplementary Movie 5 ). The apical surface of the epithelium is displaced in the basal direction, while the basal surface moves in the opposite direction ( Fig. 4b,d,f ). This movement of the luminal surface occurs in parallel with the mitotic rounding of the cell, expanding the lumen locally (space to left of white line in Fig. 4b ). As the width of the cell increases and the height of the cell body decreases, the contraction proceeds ( Fig. 4b,e ; change in ab length at maximal contraction=−4.33±0.47 μm, n =12 cells; see Supplementary Fig. 4 for other contraction examples). Since the cell is mechanically coupled to the surrounding epithelium by its basal attachment and their apical junctions with the neighbouring cells ( Fig. 4g ), it seems that ab cell shortening leads to a reduction in ab length of the epithelium ( Fig. 4d,e ). We observed that when remodelling of the basal attachment to a thin basal process linked to the rounded cell is completed (arrow in Fig. 4g ), the contraction of the epithelium diminishes ( Fig. 4e,f ). Then, the cell continues rounding until completion, although the epithelium would no longer be so tightly coupled to changes in cell shape ( Fig. 4e,f ). Finally, a net decrease in ab epithelial length is obtained after the entire mitotic process (change in ab length at postmitotic compared to premitotic=−2.13±0.10 μm, 45-min period). Different from the epithelial thinning process described above, these ab contraction events occur in individual mitotic cells. While, the thinning is a long-term process that takes 6 h to reduce the thickness of the medial epithelium by 9 μm, the mitotic contraction is a rapid event able to produce a transient 7 μm reduction in 12 min, which finally results in a stable reduction of about 2 μm ( Fig. 4e,f ). These observations show that small areas of the epithelium contract in a way that is spatiotemporally coordinated with the shortening of the mitotic cell, and suggest that the rounding cell could generate a pulling force on the luminal wall that increases the intraluminal space. 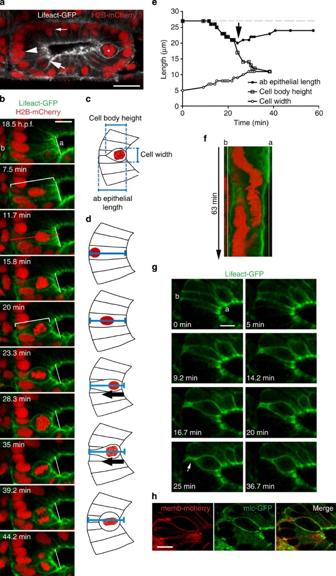Figure 4: Mitotic cell rounding and epithelial contraction during lumen expansion. (a) Cells at different stages of INM. Arrowhead points to a cell with nucleus in the basal position. The small arrow shows a nucleus migrating towards the apical domain. The asterisk marks a mitotic rounded cell positioned in the apical domain. The big arrow points to a cell segregating their chromosomes. Scale bar, 20 μm. (b) Selected planes from a high temporal resolution movie of a mitotic cell rounding event and the associated epithelial contraction. The white line indicates the position of the luminal wall of the epithelium before rounding begins. The red line indicates the region used to build the kymograph show inf. The white brackets show the ab epithelial length before (18.5 h.p.f.) and during rounding (20 min). In the second panel, the minutes elapsed from the first panel are shown. Scale bar, 10 μm. (c) Schematic representation of the lengths plotted ine. ab, apicobasal. (d) Schematic representation of the mitotic cell rounding and pulling event. As the cell increases in width, the ab epithelial length of the tissue decreases. The blue segment represents the ab epithelial length at the starting point. The black arrows indicate the period when the pulling occurs. (e) Quantification of the cell and tissue dimensions from the movie showed inb. The arrow indicates the moment when contraction stops while the cell continues rounding. The dashed line indicates the initial ab epithelial length. (f) Kymograph of the rounding-associated contraction shown inb. The red line shown inbindicates the region used to build the kymograph. (g) Selected planes of a movie showing the basal process remodelling during cell rounding. The signal of Lifeact-GFP increases in the basal domain (9.2 min) when rounding begins. Then, during rounding the basal attachment is remodelled (from 14.2 to 20 min) until the basal process (arrow) is established (from 25 min). Scale bar, 10 μm. The embryos are Tg(actb1:lifeact-GFP). (a: apical, b: basal). (h) mlc-GFP localization (green) during a contraction event associated with mitotic cell rounding. The embryos are Tg(β-actin:myl12.1-eGFP) and express memb-mCherry. Scale bar, 10 μm. Figure 4: Mitotic cell rounding and epithelial contraction during lumen expansion. ( a ) Cells at different stages of INM. Arrowhead points to a cell with nucleus in the basal position. The small arrow shows a nucleus migrating towards the apical domain. The asterisk marks a mitotic rounded cell positioned in the apical domain. The big arrow points to a cell segregating their chromosomes. Scale bar, 20 μm. ( b ) Selected planes from a high temporal resolution movie of a mitotic cell rounding event and the associated epithelial contraction. The white line indicates the position of the luminal wall of the epithelium before rounding begins. The red line indicates the region used to build the kymograph show in f . The white brackets show the ab epithelial length before (18.5 h.p.f.) and during rounding (20 min). In the second panel, the minutes elapsed from the first panel are shown. Scale bar, 10 μm. ( c ) Schematic representation of the lengths plotted in e . ab, apicobasal. ( d ) Schematic representation of the mitotic cell rounding and pulling event. As the cell increases in width, the ab epithelial length of the tissue decreases. The blue segment represents the ab epithelial length at the starting point. The black arrows indicate the period when the pulling occurs. ( e ) Quantification of the cell and tissue dimensions from the movie showed in b . The arrow indicates the moment when contraction stops while the cell continues rounding. The dashed line indicates the initial ab epithelial length. ( f ) Kymograph of the rounding-associated contraction shown in b . The red line shown in b indicates the region used to build the kymograph. ( g ) Selected planes of a movie showing the basal process remodelling during cell rounding. The signal of Lifeact-GFP increases in the basal domain (9.2 min) when rounding begins. Then, during rounding the basal attachment is remodelled (from 14.2 to 20 min) until the basal process (arrow) is established (from 25 min). Scale bar, 10 μm. The embryos are Tg(actb1:lifeact-GFP). (a: apical, b: basal). ( h ) mlc-GFP localization (green) during a contraction event associated with mitotic cell rounding. The embryos are Tg(β-actin:myl12.1-eGFP) and express memb-mCherry. Scale bar, 10 μm. Full size image Mitotic rounding cells pull the luminal surface Imaging of the rounding cells indicates a putative mechanical role on lumen expansion. We observed that during the rounding process, F-actin levels increase throughout the cellular cortex ( Fig. 4b and Supplementary Movie 5 , distinct from the enrichment observed in the apical domain in all cells of the vesicle, see Fig. 1 ). Live imaging of myosin light-chain GFP indicates that actomyosin flows also occur in the cell cortex ( Fig. 4h and Supplementary Movie 6 ). An actomyosin cortex is present in rounded cells in many systems and it is important for the changes in cell shape during mitotic rounding [25] . In the otic epithelium, the actomyosin cortex may underlie the ab shortening during rounding and, given the attachment between the rounding cell and their epithelial neighbours, this could generate the force that contracts the epithelium. To test if a single rounding cell exerts a force on the epithelium, we performed laser microsurgery experiments that allowed us to mechanically characterize the cell–tissue interactions in vivo . First, we performed subcellular laser severing (that is, without inducing cell lysis) of the actomyosin cortex to analyse the tension present in the cell. When we make a laser cut in the lateral domain of the actin cortex of a rounding cell, a bleb grows during the retraction of the two ablated ends ( Fig. 5a,a′ ; Supplementary Movie 7 ). Then, F-actin is recruited to the cortex of the bleb in a kind of ‘healing’ response of the cytoskeleton, and the bleb retracts ( Supplementary Movie 7 ). Bleb formation was previously related to cortical actomyosin tension [26] . The observed blebs induced by cortex surgery are similar to those described in vitro for rounded cells cultured in suspension and for zebrafish primordial germ cells migrating in vivo ; they were shown to be generated by a break in the actin cortex in cells with increased intracellular hydrostatic pressure [26] , [27] . Remarkably, in the otic vesicle, the rounding cells are immersed in a packed epithelium, such that the rounding severed cells are pushing over other cells to form the bleb. This also suggests that the rounding cells have a higher intracellular hydrostatic pressure than neighbouring ones. Both retraction of the actin mesh and formation of a bleb when the cortex is severed indicate that the cell is under mechanical tension. To evaluate the magnitude of this tension, we took advantage of the fact that some interphase cells also show a faint but detectable F-actin signal in their cortex, which enabled us to perform laser cuts. When we severed the cortex of these cells, a bleb did not form but a smaller retraction was observed, indicating that not only the rounding cells are under tension ( Fig. 5b,b′ ; Supplementary Movie 8 ). We then estimated the initial recoil velocity of the F-actin cortex as a quantitative estimate of tension in the network [28] , [29] , [30] . The recoil velocity in the rounding cells was higher than that in the interphase cells ( Fig. 5c ), indicating that rounding cells produce higher tension in their cortical mesh. These experiments suggest that increased cortical tension in the rounding cells could mediate the contraction of the epithelium. 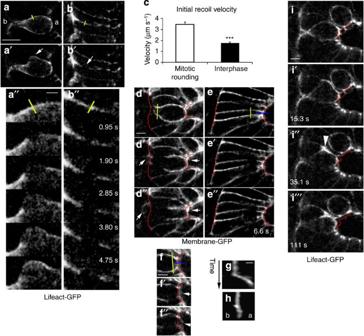Figure 5: Mitotic rounding cells pull the epithelial walls. (a–a′′ andb–b′′) Laser microsurgery of the actin cortex in the lateral membrane of a mitotic rounding (a–a′′) or an interphase cell (b–b′′). (a–a′ andb–b′) Images before (a,b) and after (a′,b′) cut showing the bleb (a′) or the hole (b′) produced during recoil of the actin cortex (arrows). (a′′,b′′) High magnification of cortical dynamics after cut. (c) Initial recoil velocities for mitotic rounding and interphase cells. Data are mean±s.e.m. (n=12, 12 embryos),t-test, ***P<0.0001. (d–d′′) Laser ablation of the plasma membrane in a rounding cell. (d) Image before ablation. (d′,d′′) The arrows point to the displacement of the apical and basal walls of the epithelium (the red lines illustrate their position before ablation). In (e–e′′), the same experiment asdbut in a cell in interphase. (f–f′′) Detail of laser ablation of the lateral plasma membranes close to the apical domain in a rounding cell before (f) and after ablation (f′,f′′). The times of the images are the same as ine–e′′. (g,h) Kymographs generated from the bars shown in blue infande, respectively. (i–i′′′) Pulling behaviour produced by accumulation of actin in the lateral membrane (white arrowhead,i′′) after cortex was severed in a rounding cell. The red line shows the position of the luminal wall before the cut (i), which remains in the same position until actin recruitment (i′). (i′′) The apical pulling begins and intraluminal space is rapidly generated between the red line and the luminal wall (i′′′). This wall displaces asymmetrically, enhanced on the lateral side where actin accumulates (i′′′). a, apical, b, basal. The yellow lines show the track of the ablation laser. The signals are Lifeact-GFP ina,b,i, and memb-GFP ind–h. Time after laser cuts are indicated. Magnification bars: 10 μm ina,b; 2 μm ina′,b′; 5 μm ind–f,iand 1 μm ing,h. Figure 5: Mitotic rounding cells pull the epithelial walls. ( a – a ′′ and b – b ′′) Laser microsurgery of the actin cortex in the lateral membrane of a mitotic rounding ( a – a ′′) or an interphase cell ( b – b ′′). ( a – a ′ and b – b ′) Images before ( a , b ) and after ( a ′, b ′) cut showing the bleb ( a ′) or the hole ( b ′) produced during recoil of the actin cortex (arrows). ( a ′′, b ′′) High magnification of cortical dynamics after cut. ( c ) Initial recoil velocities for mitotic rounding and interphase cells. Data are mean±s.e.m. ( n =12, 12 embryos), t -test, *** P <0.0001. ( d – d ′′) Laser ablation of the plasma membrane in a rounding cell. ( d ) Image before ablation. ( d ′, d ′′) The arrows point to the displacement of the apical and basal walls of the epithelium (the red lines illustrate their position before ablation). In ( e – e ′′), the same experiment as d but in a cell in interphase. ( f – f ′′) Detail of laser ablation of the lateral plasma membranes close to the apical domain in a rounding cell before ( f ) and after ablation ( f ′, f ′′). The times of the images are the same as in e – e ′′. ( g , h ) Kymographs generated from the bars shown in blue in f and e , respectively. ( i – i ′′′) Pulling behaviour produced by accumulation of actin in the lateral membrane (white arrowhead, i ′′) after cortex was severed in a rounding cell. The red line shows the position of the luminal wall before the cut ( i ), which remains in the same position until actin recruitment ( i ′). ( i ′′) The apical pulling begins and intraluminal space is rapidly generated between the red line and the luminal wall ( i ′′′). This wall displaces asymmetrically, enhanced on the lateral side where actin accumulates ( i ′′′). a, apical, b, basal. The yellow lines show the track of the ablation laser. The signals are Lifeact-GFP in a , b , i , and memb-GFP in d – h . Time after laser cuts are indicated. Magnification bars: 10 μm in a , b ; 2 μm in a ′, b ′; 5 μm in d – f , i and 1 μm in g , h . Full size image Next, we directly evaluated whether the cell is indeed pulling on the epithelial walls by performing cell ablation (that is, laser-induced cell lysis targeted to the membrane), thus breaking the hypothetical mechanical coupling between the rounding cell and the epithelial surfaces. If the rounding cell deforms the tissue by applying pulling forces, we expected that cutting it would release the contraction, and thus the apical and basal epithelial walls would move apart in opposite directions. Figure 5d,d′ and Supplementary Movie 9 show that this is the case when we ablate a rounding cell close to the basal domain. Ablation in a subapical region produced even stronger movements of the luminal membrane ( Fig. 5f,f′ ). In contrast, ablation of cells in interphase does not produce displacement of the epithelial walls ( Fig. 5e,e′ ; Supplementary Movie 10 ). Taken together, these experiments demonstrate that the rounding cell drives contraction of the epithelium by pulling on the epithelial walls during ab shortening. They also suggest that cortical tension in the actomyosin cortex accounts for this contraction. Thus, the rounding cell exerts a force on the luminal wall able to increase the luminal space. We analysed the ‘healing’ response that occurred after severing the cortex and observed that the dramatic and rapid recruitment of actin to the site after cut induces pulling forces on the apical surface of the lumen within seconds ( Fig. 5i–i′′′ ; Supplementary Movie 11 ). This damage-induced contractile behaviour shows that cortical actin accumulation in the lateral membrane of the cell is associated with deformation of the tissue with much faster dynamics than the time required to add new apical membrane (this damage-induced pulling occurs in seconds, while the endogenous process takes minutes). This also demonstrates that a local increase in luminal volume by cell pulling is mechanically possible in this epithelium, supporting the proposed role for the rounding cell. Mitotic cell rounding accelerates lumen expansion To evaluate if mitotic cell rounding is indeed contributing to lumen expansion, we decided to arrest the cell cycle at different phases ( Fig. 6a ). First, we blocked the S-phase using the same combination of AH as described above. This treatment inhibited all the mitotic phases, including initial nuclear apical migration ( Supplementary Movie 12 ). AH inhibition during the lumen expansion phase led to smaller lumens ( Fig. 6b,c ), caused by a reduction in volume expansion kinetics (volume expansion rate, DMSO=4.77±0.42 × 10 3 μm 3 h −1 , AH=2.79±0.37 × 10 3 μm 3 h −1 ; Fig. 6g ). Interestingly, while expansion in the AP axis was reduced, that of the ML was not affected (axis expansion rate, AP DMSO=1.91±0.08 μm h −1 , AP AH=0.42±0.22 μm h −1 , ML DMSO=3.17±0.17 μm h −1 , ML AH=3.04±0.45 μm h −1 ; Fig. 6h and Supplementary Fig. 6b ). This experiment demonstrates the relevance of mitosis for lumen expansion, particularly along the AP axis. 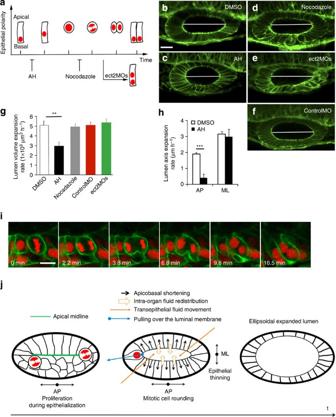Figure 6: Mitotic cell rounding contributes to lumen expansion. (a) Diagram of the effect of the various experimental approaches on the progression of the INM and cell division events. (b–f) Vesicles at 22 h.p.f. after lumen expansion from wt (b–d),ect2morphant (e) or controlMO-injected (f) embryos mounted from 19 to 22 h.p.f. with DMSO (b,e,f), AH (c) or nocodazole (d). Memb-GFP (c,e) and Lifeact-GFP (b,d,f) are shown in green. Scale bar, 20 μm. (g) Quantification of lumen volume expansion rate from 19 to 22 h.p.f. from the experimental groups indicated. Data are mean±s.e.m. (n=5 embryos). ANOVA **P<0.01. (h) Quantification of lumen axis expansion rate from 19 to 22 h.p.f. in DMSO- and AH-treated embryos. Data are mean±s.e.m. (n=5 embryos),t-test ***P<0.001. (i) Selected planes from a high temporal resolution movie of a mitotic cell during lumen expansion from anect2morphant embryo showing a binucleated cell after impaired cytokinesis. Injection of embryos with the controlMO did not produce a cytokinesis phenotype. memb-GFP is shown in green and H2B-mCherry in red. Scale bar, 10 μm. (j) Proposed model for the mechanisms involved in shaping the lumen of the otic vesicle. Figure 6: Mitotic cell rounding contributes to lumen expansion. ( a ) Diagram of the effect of the various experimental approaches on the progression of the INM and cell division events. ( b – f ) Vesicles at 22 h.p.f. after lumen expansion from wt ( b – d ), ect2 morphant ( e ) or controlMO-injected ( f ) embryos mounted from 19 to 22 h.p.f. with DMSO ( b , e , f ), AH ( c ) or nocodazole ( d ). Memb-GFP ( c , e ) and Lifeact-GFP ( b , d , f ) are shown in green. Scale bar, 20 μm. ( g ) Quantification of lumen volume expansion rate from 19 to 22 h.p.f. from the experimental groups indicated. Data are mean±s.e.m. ( n =5 embryos). ANOVA ** P <0.01. ( h ) Quantification of lumen axis expansion rate from 19 to 22 h.p.f. in DMSO- and AH-treated embryos. Data are mean±s.e.m. ( n =5 embryos), t -test *** P <0.001. ( i ) Selected planes from a high temporal resolution movie of a mitotic cell during lumen expansion from an ect2 morphant embryo showing a binucleated cell after impaired cytokinesis. Injection of embryos with the controlMO did not produce a cytokinesis phenotype. memb-GFP is shown in green and H2B-mCherry in red. Scale bar, 10 μm. ( j ) Proposed model for the mechanisms involved in shaping the lumen of the otic vesicle. Full size image The results of AH blockade indicate that some of the events occurring once the nucleus starts to migrate are important for the expansion process. To test if cell rounding is the key event, we then blocked mitosis immediately after rounding. In this way, if mitotic rounding is sufficient to facilitate expansion, the growth of the lumen should proceed normally in this condition. We blocked the cell cycle by using nocodazole, a microtubule polymerization inhibitor. Similar to the effect of other inhibitors as colchicine [31] , nocodazole at low doses (0.1 μg ml −1 ) inhibits specifically the chromosome segregation and cytokinesis, arresting the cells in the mitotic rounded stage ( Fig. 6a ) [32] . In our experiments, nocodazole treatment did not affect the general morphology of the cells during expansion, but led to apical accumulation of mitotic rounded cells over time ( Supplementary Movie 13 ). In contrast to the effect of AH, the kinetics of lumen volume expansion were not affected by nocodazole (volume expansion rate, nocodazole=4.66±0.24 × 10 3 μm 3 h −1 , see control value above; Fig. 6d,g and Supplementary Fig. 6b ), which supports the hypothesis that mitotic cell rounding is key for expansion and suggests that the later phases of mitosis are not relevant in these time frames. To confirm the relevance of cell rounding by other means, we next used a genetic approach. The guanine exchange factor Ect2 is a well-known activator of small GTPases (such as Rho), essential for cytokinesis in Drosophila and cultured cells [33] , [34] , although this role has not yet been analysed during zebrafish development. We hypothesized that a blockade of ect2 in our system would also inhibit cytokinesis, allowing us to evaluate whether the mitotic phases that occur after or before this process play a role during expansion. We injected ect2 MOs, disturbing splicing of the ect2 pre-mRNA ( Supplementary Fig. 5 ). Before 24 h.p.f., the general morphology of the otic vesicle was not affected by the ect2 MOs, nor was the general development of the embryos (at later stages, some neural defects appeared). However, cytokinesis was perturbed in the otic vesicle epithelium (95±1% of cytokinesis events inhibited, Fig. 6i ; Supplementary Movie 14 ). While the nucleus migrates to the apical domain and the chromosomes segregate, the cleavage furrow does not proceed and binucleated cells appear ( Fig. 6i ). We could not detect any other cellular defect and the cell rounding proceeds normally. When we measured lumen expansion kinetics in the ect2 MOs-injected embryos, we found similar values than in controlMO embryos (volume expansion kinetics, controlMO=4.80±0.29 × 10 3 μm 3 h −1 , ect2 MOs=5.06±0.32 × 10 3 μm 3 h −1 ; Fig. 6e,f,g and Supplementary Fig. 6b ), indicating that cytokinesis is not essential for expansion, and once more supporting the preceding rounding as the important event. We also analysed the Tg hi3820 embryos ( ect2 mutant), which have an identical cytokinesis phenotype to that observed in the morphant embryos ( Supplementary Fig. 6a ). However, in these embryos, the early stages of lumen formation are affected, precluding their use for analysing expansion kinetics. In summary, these experiments suggest that mitotic cell rounding accelerates lumen expansion in the inner ear. In this study, we imaged and quantified for the first time the dynamics of the zebrafish inner ear hollowing. The geometrical features of the otic vesicle lumen, its small size and the fact that it is a closed cavity (not a tube), allowed us to analyse the organ as a whole, which is not possible in vivo with other vertebrate hollowed model organs, such as the brain ventricle or the gut. This approach revealed essential morphogenetic processes for lumen growth and shape that had not been detected previously. First, epithelialization of the placode organizes the apical surface from where the lumen will develop, predetermining the gross size of the luminal AP axis ( Fig. 6j ). Second, ML axis expansion seems to be controlled by an active role of the epithelial cells, which shrink and secrete fluid to the lumen. Simultaneously with these long-term cell-shortening events, the length of the AP axis is adjusted during expansion by a tissue contraction mechanism driven by cell shortening caused by mitotic cell rounding events. Thus, all these mechanisms are coordinated spatiotemporally to mould the shape of the expanding cavity ( Fig. 6j ). Little is known about the biomechanics underlying lumen growth. In the brain ventricle, actomyosin-dependent relaxation of the epithelium is required to expand the lumen [35] . During Drosophila tracheal development, forces from tip migratory cells stimulate cell intercalation to elongate the tube [6] . This is an example of forces indirectly promoting lumen growth by increasing the number of cells belonging to the tube. Here we propose that contraction driven by mitotic rounding works as a mechanical force to deform the tissue along the AP axis, thus favouring intraluminal fluid accumulation. Once the tension is decreased after rounding, the lumen is bigger along this axis. This would represent an example of direct forces operating over the luminal membrane, uncovering a new mechanical mechanism for cavity expansion. The mechanical effect of mitotic cell rounding is probably reinforced by the ingress of fluid into the cavity that maintains the hydrostatic pressure. A related mechanical role for mitotic cell rounding during tracheal placode invagination has also been identified in Drosophila [31] . In this case, the cell rounding event does not directly exert a force over the tissue but releases the tension on apically constricted neighbouring cells, accelerating the invagination process. To our knowledge, our work shows, for the first time in vertebrates, both a mechanical role for mitotic cell rounding and the direct role of a cellular mechanical input in expanding a cavity. The mechanics of mitotic cell rounding has been analysed in cultured cells [36] . Laser ablation was used to analyse in vivo the forces generated by actomyosin structures organized in apical layers or cables [29] , [37] , [38] . Only a few studies have focused on the cortical actomyosin mesh of rounded cells, but these were done in cultured cells or in vivo -isolated cells, and none were done in mitotic cells [26] , [39] . Here we used laser microsurgery to analyse the mechanics of mitotic rounding cells in the context of a vertebrate epithelium. In concordance with the demonstration that a rounded cell can exert forces against other structures in vitro [36] , we observed a related behaviour in vivo , with changes in shape occurring during rounding, exerting pulling forces on the tissue. This constitutes a direct mechanical action of a single-cell deforming an epithelium. Similar to the actomyosin requirement to round when a cultured cell adheres to the substrate [36] , we propose that the actomyosin cortex in the rounding cell pulls the epithelial walls as a consequence of its connections with the surrounding cells. Moreover, the bleb formed after laser severing also highlights the importance of both intracellular hydrostatic pressure and the actomyosin cortex during rounding in vivo in an epithelial context, whose interplay was previously shown to be required for rounding in vitro [36] . On top of these intrinsic otic forces, surrounding tissues could also provide mechanical constraints and impinge on the otic vesicle and lumen shape, a question that still needs to be addressed. While we cannot discard a long-term contribution of cell division to expand the lumen by adding cells to the tissue, as occurs in other models [4] , this does not seem to be the case in the otic vesicle in the time frame analysed. The AP expansion does not require the cell division process per se but only the early mitotic events (cell rounding-associated shortening). Moreover, all the cell cycle inhibitors tested (AH, nocodazole and ect2 MOs) interfere to a similar extent with the increase in the number of cells forming the luminal surface of the cavity ( Supplementary Fig. 6c ), but only the AH treatment, which affects cell rounding, reduces the expansion kinetics. We propose here that gain of luminal fluid at the expense of epithelial volume is an essential part of the lumen growth, which highlights the presence of a specific morphogenetic process occurring in the epithelium, rather than simply a fluid transportation function from outside the organ. We demonstrate that this process requires the atp1a1 gene, while putative channels and transporters involved can be speculated from reported gene expression data ( Supplementary Note 1 ). We also show that epithelial thinning occurs during brain ventricle expansion and, while not reported, we also observe this in published images of other lumen forming systems (gut and Kuppfer vesicle [5] , [23] ). This suggests that epithelial thinning is a widespread driver of lumen growth and shape beyond the inner ear cavity. In addition to the intra-organ fluid redistribution, it is also possible that fluid lost by epithelial cells move outside of the organ. In this case, the thinning of the epithelium would contribute to lumen morphogenesis mainly by releasing space from the vesicle to be filled with fluids. The nature of the signal that triggers remodelling of the epithelial cells during expansion is still unknown. One possibility is a biological signal, such as a factor secreted from surrounding tissues or an activation of transcription factors cell autonomously. Alternatively, a mechanical signal could be involved. Similar to ab shortening of the otic vesicle cells observed here, follicle cells from the Drosophila ovary, flatten concomitantly with cyst growth by a mechanism dependent on intracyst fluid pressure and cell adhesion remodelling [40] , although the contribution of cell flattening for cyst growth was not evaluated. Thus, it is possible that cell shortening events in otic vesicle cells are also the consequence of an initial increase in intraluminal fluid pressure. Several zebrafish mutants (mib, ace and pan, carrying mutations in genes involved in Notch and fibroblast growth factor pathways and transcriptional elongation, respectively) display smaller spherical otic vesicle lumens rather than biaxial ellipsoidal ones [41] , [42] , [43] similar to the emi1 morphant embryos. These similarities may highlight the underlying processes affected in these mutants, which probably involve placode induction or early proliferation defects. The development of mechanisms that regulate size, shape and positioning of cavities is relevant for the proper functioning of organs. Here we highlight the relevance of epithelial cells in actively contributing to lumen growth beyond their classical role in introducing fluids from outside of the organ or adding new cellular blocks to the epithelial wall. Either by concerted cell remodelling that thins the tissue or by individual tension applied to the luminal membrane, these two mechanisms provide a new perspective of our understanding of lumen construction. Thus, the interplay between mechanics and hydrodynamics regulates lumen shape, which has important implications for lumen morphogenesis and its associated pathologies. Zebrafish AB wild-type zebrafish strain, transgenic lines expressing Lifeact-GFP (Tg(actb1:lifeact-GFP)), Utrophin-GFP (Tg(actb1:GFP-utrCH)) [20] and Myosin light-chain GFP (Tg(β-actin:myl12.1-eGFP)) [20] , and the hi3820Tg ect2 mutant line [44] , [45] were maintained and bred according to the standard procedures [46] at the aquatic facility of Parc de Recerca Biomèdica de Barcelona (PRBB). All experiments conform to the guidelines from the European Community Directive and Spanish legislation for the experimental use of animals. Microinjection and drug treatments To label cellular and subcellular structures, mRNAs encoding the following fusion proteins were injected at one-cell stage after being synthetized with the SP6 mMessenger mMachine kit (Ambion): H2B-mCherry or H2B-GFP (100–150 pg) [47] , Pard3-GFP or Pard3-RFP (50–75 pg) [48] , [49] , Lyn-EGFP (membrane-GFP 100–150 pg) [50] , membrane-mCherry (100–150 pg) [51] , Lifeact-RFP or Lifeact-GFP (150 pg) [52] , hZO1-GFP (100 pg) [53] , GFP and Kaede (50 pg) [54] . To interfere with endogenous expression, embryos were injected at one-cell stage with 1.6 ng per embryo of emi1 translation blocking morpholino (5′- GTAGTTTGGACACTTCATATTGAGG -3′) (ref. 21 ), 6 ng per embryo of atp1a1 splice site (exon 5–intron 6) blocking morpholino, (5′- AATATAATATCAATAAGTACCTGGG -3′) (ref. 24 ), 1.6, 4 or 6 ng per embryo of standard control morpholino (5′- CCTCTTACCTCAGTTACAATTTATA -3′) or a combination of 4 ng per embryo of each ect2 splice blocking morpholinos designed according to the manufacturer’s recommendations (Gene Tools, LLC). The sequences of the ect2 morpholinos used are: ect2 MO1 (targeted to the exon3-intron3 junction), 5′- TCTTTCTAACAGTACCTGAAGAGCT -3′ and ect2 MO2 (targeted to intron6-exon7 junction), 5′- GCAACCTGCACAGAAATAAACTCGT -3′. Ect2 splicing morpholinos were tested for their efficiency in splicing using reverse transcription-PCR (primers used: ect2F2 (5′- TCATTGGTCTACACTCAGACG -3′), ect2F6 (5′- CTCAACTTGTCCCTCTGCTTC -3′), ect2R8 (5′- CTCTGTGCTCCCATGCCTTG -3′) and ect2R5 (5′- AGGATACGGCTGTCATTCTTG -3′). Ouabain treatment was performed in embryo medium over dechorionated embryos for the times indicated. For experiments measuring lumen expansion rate, nocodazole 0.1 μg ml −1 (Sigma), aphidicolin 300 μM (Merck) in combination with hydroxyurea 100 mM (Sigma) or DMSO (Sigma) were added to the agarose mounting media. Each embryo was imaged several times at different time points during development. Of all nocodazole-treated embryos, lumen expansion was analysed only in those in which mitotic rounding cells accumulated in the apical domain of the otic vesicle, while most of the other cells had normal morphology. Ect2 MOs-injected embryos were also mounted with DMSO and imaged sequentially. Early treatments with AH (between 10 and 14 h.p.f.) were performed in embryo medium over dechorionated embryos. At 14 h.p.f., the AH was washed out by replacing the embryo medium with fresh embryo medium several times, then incubated for several hours before being mounted and imaged. Morphological analysis of morphant embryos To confirm the previously identified emi1 morphant phenotype [21] (injection of emi1 MO was used instead of the emi1 mutant line to address whether early defects in the length of the apical midline have consequences on the AP length of the lumen at later stages, given that mitosis is also affected during the expansion stages in the mutant [21] ), emi1 MO-injected embryos were evaluated for the number of cell division events in the otic epithelium by manual quantification of the chromosome segregation events in movies of H2B-mCherry injected embryos. For the analysis of lumen shape and size dynamics in the morphants, only embryos with a curved tail or those with vesicles with a reduced number of cells (depending on the stage analysed) were used for quantification. Ect2 MOs-injected embryos were time-lapse imaged to detect cytokinesis defects, and the number of inhibited events was quantified using the FIJI cell counter plugin (Kurt De Vos, University of Sheffield). The ect2 MOs were titrated to determine the concentration required to prevent toxicity and observe cytokinesis defects. Injection of 4, 2 or 0.4 ng per embryo of each ect2 MO led to about 87.5% (21/24), 57% (12/21) and 0% (0/29) of embryos with affected cytokinesis, respectively (higher concentrations also led to a higher percentage of abnormal events in every affected embryo). To describe the cellular phenotype in detail, live imaging was performed at high temporal resolution (see below). For the analysis of lumen expansion rate, only embryos with binucleated cells in the otic epithelium were used. In the atp1a1 MO experiments, we observed the same defects in the brain ventricle lumen that were reported previously [24] . Live imaging and data analysis Live embryos were embedded in 1% low melting point agarose in embryo medium with tricaine (150 mg l −1 ) for dorsal confocal imaging using a × 20 (0.8 NA) glycerol-immersion lens. Imaging was performed using a SP5 Leica confocal microscope in a chamber heated to 28.5 °C. Twenty to 80-μm-thick z -stacks spanning the entire or a portion of the otic vesicle (a z -plane imaged every 0.5–2 μm) were taken every 5–20 min for 2-12 h. For high temporal resolution, sections were acquired every 40–120 s. Raw data were analysed and quantified using FIJI software [55] . Before quantifications, all z -stacks were aligned in 3D to correct for variability in orientation during mounting, to guarantee the coronal sectioning of the vesicle. Measurements of vesicle or lumen axis length were performed on the largest coronal, sagittal or transverse planes of the structure, measuring the longest distance between the outer borders in each axis. To calculate volume, the x–y area of the structure in each plane of the z -stack was measured and then multiplied by the z spacing between planes. To calculate expansion rates, the lengths of the axes or volumes were calculated at sequential time points for the same mounted embryo. Then, a linear regression of the measured values over time was fit. The initial stage of the embryo was determined not only by phenotypic characterization, but once mounted, only the embryos with initial lumen volume of 3–5 × 10 3 μm 3 were used to calculate expansion rates. To follow the dynamics of cell dimensions, the length of the lateral (ab length) or apical membrane (distance between two cell junctions) was measured at different sequential time points in every mounted embryo. Several cells from the coronal plane with the largest lumen area were analysed, all at or surrounding the four vertices of the vesicle (A, P, L and M). To analyse cell and epithelium shape changes during mitotic cell rounding events, acquisition was performed every 40 s in several z -planes, to facilitate detection of the contraction. The number and magnitude of contraction events identified are underestimated, as some of them occur in distinct 3D orientations from the imaged plane. Movies were assembled by selecting the plane with the highest lumen area (or better visualization of the apical stripe) from every z -stack at every time point, thus manually correcting for z movement of the structure during development (in the contraction events analysis, this correction was not performed to avoid manually introducing artifacts into the changes in epithelial length; since these experiments were brief, z movement does not seem to make a significant contribution to the process). To construct the kymographs, a region from a time-lapse of one z -plane was resliced with FIJI, following the signal in the region selected over time. To quantify the number of cell divisions in the otic epithelium, higher temporal resolution videos (1 min frequency) in 4D from the period of time indicated were analysed manually to detect every chromosome segregation event. Representative panels displaying the plane with the highest lumen or placode area from a z -stack were used to prepare the figures. Single cell 3D reconstruction and volume quantification Embryos were injected in the yolk at the one-cell stage with Pard3-RFP and H2B-mCherry mRNA to uniformly stain the luminal surface and the nucleus of the cells. At the 16–32-cell stage, GFP mRNA was injected into one cell of the same embryos to generate mosaic embryos bearing only a few isolated cells with cytosolic fluorescence. At 17 h.p.f., the otic vesicle was imaged at high 3D resolution (0.5 μm z distance between planes). Stained cells located in different regions of the vesicle were tracked over time and imaged at different time points until 23 h.p.f. To isolate the data of the analysed cell, the acquired images were cropped in 3D using the 3D viewer plugin [56] of FIJI. To reconstruct the 3D shape and quantify the volume of every cell, the surface function of the Imaris software (Bitplane) was applied to the z -stack. Pard3 staining was used to monitor the size of the lumen and the nuclear staining allowed us to ensure volume quantification of single cells. In some experiments, the Kaede protein was used (instead of GFP) and photoconverted with an ultraviolet laser at 17 h.p.f. (before the first 3D imaging). This allowed us to track only one photoconverted cell in every vesicle (in this case, a H2B-GFP protein was used to stain the nucleus), to be sure that we were imaging the same cell at different time points. Both cytosolic proteins produced identical results. Laser ablation experiments The laser microsurgery experiments were performed on a custom system described previously [57] . In brief, a 355-nm 470-ps pulsed laser is coupled and scanned into an inverted microscope (Axiovert200M, Carl Zeiss, Germany) and imaged with a CCD ORCA camera (Hamamatsu). Basic optical sectioning is achieved using a custom spinning disk unit working with one 488 nm laser line. To achieve intracellular severing, pulses energy was between 150 and 250 nJ. Cell disruption was performed at 300–500 nJ per pulse. Both types of experiment were performed by scanning the beam along a line of variable length and with about five pulses per micron density. To image and cut the F-actin cortex, wild-type embryos were injected with Lifeact-GFP mRNA at the 1- or 16–32-cell stage (mosaic staining for improved contrasted of the cortex of a single cell), or Tg(actb1:lifeact-GFP) embryos were used. For cellular ablation of the membrane, we used embryos injected at the one-cell stage with Lyn-GFP mRNA. The embryos were mounted at 19–21 h.p.f. and live imaged until a rounding cell was detected. Image acquisition was performed at 0.9–0.95 s per frame. In the cortex-severing experiments, the power of the laser was calibrated to avoid irreversibly damaging the cell. Imaging for several minutes after the cut confirmed that cortex-severed cells survive, recover their normal shape and divide normally. Moreover, none of the cortex-severed cells used for subsequent analysis showed release of the non-cortical cytosolic Lifeact-GFP to the outside of the cell, a hallmark of membrane broken cells. Recoil velocities were quantified directly over the image sequences by measuring the retraction displacements with FIJI at the first time frame following the cut. In the cell ablation experiments, we simultaneously ablated the two lateral plasma membranes of the targeted cell, to disturb its ab integrity. In more apically localized ablations, the apical wall is preferentially displaced over the basal one. In contrast, basal ablations of the lateral membrane led to more movement in the basal than in apical epithelial surfaces. Kymographs were generated using a custom macro (author: Jens Rietdorf). Statistics All statistical comparisons are indicated in the figure legends, including the unpaired Student’s t -test, one-way ANOVA (analysis of variance; Tukey post-test) and linear regression, performed using GraphPad or Microsoft Excel software. How to cite this article: Hoijman, E. et al . Mitotic cell rounding and epithelial thinning regulate lumen growth and shape. Nat. Commun. 6:7355 doi: 10.1038/ncomms8355 (2015).